Broadly tunable terahertz generation in mid-infrared quantum cascade lasers Room temperature, broadly tunable, electrically pumped semiconductor sources in the terahertz spectral range, similar in operation simplicity to diode lasers, are highly desired for applications. An emerging technology in this area are sources based on intracavity difference-frequency generation in dual-wavelength mid-infrared quantum cascade lasers. Here we report terahertz quantum cascade laser sources based on an optimized non-collinear Cherenkov difference-frequency generation scheme that demonstrates dramatic improvements in performance. Devices emitting at 4 THz display a mid-infrared-to-terahertz conversion efficiency in excess of 0.6 mW W −2 and provide nearly 0.12 mW of peak power output. Devices emitting at 2 and 3 THz fabricated on the same chip display 0.09 and 0.4 mW W −2 conversion efficiencies at room temperature, respectively. High terahertz-generation efficiency and relaxed phase-matching conditions offered by the Cherenkov scheme allowed us to demonstrate, for the first time, an external-cavity terahertz quantum cascade laser source tunable between 1.70 and 5.25 THz. Terahertz (THz, λ =30–300 μm) technology has proven that it can work in a laboratory setting, but there are few commercialized products because system-level components are large, complex and prohibitively expensive [1] , [2] . A major impediment towards widescale commercialization is the lack of an economical, compact, widely tunable mW-level THz source, particularly in 1–5 THz range. Electrically pumped semiconductor-based sources are particularly attractive because of their operating simplicity and their potential for mass production. THz quantum cascade lasers (QCLs) are a promising technology for the 1–5 THz spectral range; however, they still require cryogenic cooling to operate [3] , [4] , [5] , [6] , [7] , [8] and their tuning range is limited [9] . An alternative approach to generate THz radiation in QCLs are sources based on intracavity difference-frequency generation (DFG) in dual-wavelength mid-infrared ( λ =3–15 μm) QCLs designed to have giant optical non-linearity in the active region [10] , [11] , [12] , [13] , [14] . Not only can these sources operate at room temperature [11] , [12] , [13] , [14] , but they are also uniquely suited to provide THz output over a wide range of frequencies, as the mid-infrared frequencies in a QCL can be tuned well over 5 THz [15] , [16] and the optical non-linearity for intracavity THz DFG is not expected to change significantly over several THz of tuning [17] . The current challenge that must be addressed is their limited THz power output due to low mid-infrared-to-THz conversion efficiency. To improve THz generation efficiency, we recently proposed using a Cherenkov phase-matching scheme in THz DFG–QCLs to generate broadband difference-frequency output at an angle to the mid-infrared pumps [12] . This approach circumvents the problem of high THz absorption and inefficient THz outcoupling to free space intrinsic to THz DFG–QCLs based on collinear modal phase matching [10] , [11] , [14] . The existence of Cherenkov emission in DFG–QCLs was confirmed by us using proof-of-principle devices [12] and multimode THz generation over a 1.2 to 4.5 THz range was observed. However, these proof-of-principle devices demonstrated only a 45 μW W −2 mid-infrared-to-THz conversion efficiency, an improvement of only 5–10 times over devices based on collinear modal phase matching [10] , [11] , [14] . Similar Cherenkov devices were reported later with 50 μW W −2 conversion efficiency [13] . Here we report Cherenkov DFG devices that have been comprehensively optimized. As a result, they demonstrate record conversion efficiency in excess of 0.6 mW W −2 and record power output of nearly 0.12 mW at 4 THz at room temperature. High efficiency and relaxed phase-matching conditions of Cherenkov DFG in our devices allowed us to demonstrate, for the first time, a broadly tunable external-cavity (EC) THz QCL source, with a tuning range spanning 1.70–5.25 THz. We also demonstrate single-mode distributed feedback (DFB) THz DFG–QCL sources that provide output at 2 and 3 THz with 0.09 and 0.4 mW W −2 conversion efficiencies at room temperature, respectively. Waveguide design Cherenkov emission occurs when the phase velocity of the non-linear polarization wave in a thin slab of non-linear optical material is faster than the phase velocity of the generated radiation in the medium surrounding the slab [18] . In this case, the generated radiation is emitted at the Cherenkov angle θ C from the slab as shown in Fig. 1a . 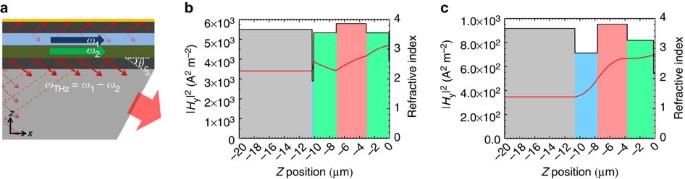Figure 1: Cherenkov waveguide geometry and mode profile. (a) Schematic of Cherenkov THz DFG in our devices. (b,c) Calculated square of H-field in the TM-polarized THz Cherenkov waves (red lines, left axes) and waveguide refractive index profiles (black lines, right axes) at 4 THz for (b) optimized devices reported here and (c) proof-of-principle devices in ref.12. For (b) and (c), the gold contact layer is positioned atz=0, cladding layers are shown in green, current injection layers in blue, active regions in red, and substrate in grey. In the case of DFG–QCLs, we can write an expression for the non-linear polarization wave at ω THz = ω 1 − ω 2 in the slab-waveguide approximation as [12] , [19] : Figure 1: Cherenkov waveguide geometry and mode profile. ( a ) Schematic of Cherenkov THz DFG in our devices. ( b , c ) Calculated square of H-field in the TM-polarized THz Cherenkov waves (red lines, left axes) and waveguide refractive index profiles (black lines, right axes) at 4 THz for ( b ) optimized devices reported here and ( c ) proof-of-principle devices in ref. 12 . For ( b ) and ( c ), the gold contact layer is positioned at z =0, cladding layers are shown in green, current injection layers in blue, active regions in red, and substrate in grey. Full size image where the z direction is normal to the QCL layers and the x direction is along the waveguide, β 1 and β 2 are the propagation constants for mid-infrared pump modes, and are z components of E -field of the mid-infrared pump modes and is the giant intersubband optical non-linearity for DFG in the QCL active region. Physically, two Cherenkov waves are generated by the non-linear polarization wave: one propagates towards the top contact and the other one towards the bottom substrate as shown in Fig. 1a . These two waves are partially reflected by various waveguide layers and may pass through the active region multiple times, and interfere with each other before finally exiting to the substrate. These effects all need to be taken into account to design an efficient Cherenkov DFG–QCL. Three major modifications were made in the structure of the current devices compared with the proof-of-principle devices in ref. 12 . First, the new devices use a 200-nm-thick InGaAs current extraction layer n-doped to 7 × 10 17 cm −3 and are separated from the active region by a 3-μm-thick layer of InP n-doped to 1.5 × 10 16 cm −3 , as opposed to a 3-μm-thick InP lower cladding and current injection layer n-doped to 10 17 cm −1 used for devices in ref. 12 . Higher electron mobility in InGaAs compared with that in InP allowed us to maintain the same, low, sheet resistance (~100 Ω/□) while using smaller-sheet doping density for the current extraction layer. Plane wave transfer matrices calculations show that the new current extraction layer have 80–90% transmission for the exiting THz Cherenkov wave at 3–4 THz, as opposed to only 20–40% transmission for the current extraction layer in ref. 12 . Second, optical non-linearity was integrated in both mid-infrared-active region stacks. This effectively doubles the interaction length of the Cherenkov wave with the non-linear material. Lastly, waveguide cladding layers thickness and doping were adjusted to provide for low THz loss and constructive interference between reflected upward and downward propagating Cherenkov waves. To observe the effect of these modifications, we modelled the Cherenkov emission as a leaky slab-waveguide mode with the propagation constant fixed at β 1 –β 2 . Our approach is based on the formalism described in ref. 20 and is generalized for the multilayer waveguide structure of our devices. The calculated squared magnitude of the H-field for the TM-polarized Cherenkov wave (| H y | 2 ) for our devices is shown in Fig. 1b along with the refractive index profile for the case of 4 THz emission. For comparison, Fig. 1c plots the same data for the non-optimized proof-of-concept devices used in ref. 12 . The simulations assumed 25-μm-wide ridge devices with mid-infrared pumps operating in TM 00 mode, each with 1.4 W of optical power propagating inside of the waveguide. Simulation results predict about ten times improvement in the Cherenkov wave intensity in the substrate compared with our proof-of-principle devices in ref. 12 , assuming the same ridge width and pump power. Band structure design The waveguide core in our devices was made up of two stacks of QCL stages designed for emission at λ 1 =8.2 μm and λ 2 =9.2 μm. Giant optical non-linearity for the DFG process is integrated in the QCL band structure by reducing the thickness of the extraction barrier and producing significant anticrossing between the lower laser level state and the injection states. As a result, the laser design effectively becomes a bound-to-continuum QCL design [21] . Details of the active region design is provided in the Methods section. The active regions were designed to have a broad mid-infrared gain bandwidth (see Supplementary Fig. 1 ) to achieve a large THz tuning range. The calculated band structure and squared moduli of the electron wave functions for one period of these structures are depicted in Fig. 2 . The design of both sections is chosen to have large optical non-linearity χ (2) for DFG between the mid-infrared pumps. Referring to the band structure described in Fig. 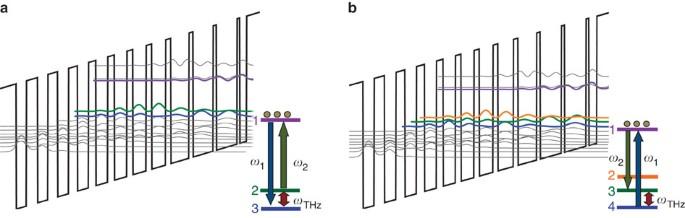Figure 2: Active region band structure. (a) Conduction band diagram for one period of active region Stack A biased at 48 kV cm−1and producing radiation around 8.20 μm. Schematic description of resonant DFG process in Stack A is shown in the bottom right. Transition dipole momentsz12=2.20 nm,z13=2.20 nm,z23=8.00 nm,E12=134.8 meV andE13=154.1 meV are calculated for this structure. Lasing atλ1occurs in near-resonance to a transition between states 1 and 3. Transition between states 1 and 2 is in near-resonance with the pump atλ2. (b) Conduction band diagram for one period of active region Stack B biased at 40 kV cm−1and producing radiation around 9.20 μm. Schematic description of resonant DFG process in Stack B is shown in the bottom right. Transition dipole momentsz12=2.00 nm,z13=2.37 nm,z14=0.60 nm,z34=9.80 nm,E12=117.0 meV,E13=134.4 meV andE14=153.6 meV are calculated for this structure. 2a , resonant intersubband optical non-linearity can be estimated using calculated energy level positions and transition dipole moments between states 1, 2 and 3: Figure 2: Active region band structure. ( a ) Conduction band diagram for one period of active region Stack A biased at 48 kV cm −1 and producing radiation around 8.20 μm. Schematic description of resonant DFG process in Stack A is shown in the bottom right. Transition dipole moments z 12 =2.20 nm, z 13 =2.20 nm, z 23 =8.00 nm, E 12 =134.8 meV and E 13 =154.1 meV are calculated for this structure. Lasing at λ 1 occurs in near-resonance to a transition between states 1 and 3. Transition between states 1 and 2 is in near-resonance with the pump at λ 2 . ( b ) Conduction band diagram for one period of active region Stack B biased at 40 kV cm −1 and producing radiation around 9.20 μm. Schematic description of resonant DFG process in Stack B is shown in the bottom right. Transition dipole moments z 12 =2.00 nm, z 13 =2.37 nm, z 14 =0.60 nm, z 34 =9.80 nm, E 12 =117.0 meV, E 13 =134.4 meV and E 14 =153.6 meV are calculated for this structure. Full size image where Δ N is the population inversion density, ez ij , ω ij and Γ ij are the dipole matrix element, frequency and broadening of the transition between states i and j. Further details describing our method for calculating the non-linearity is found in the Supplementary Note 1. For the band structure depicted in Fig. 2b , we need to account for a fourth energy level that contributes to the non-linearity and sum the non-linearity calculated using equation (1) for triplets of states 1, 2, 3 and 1, 3, 4. Assuming Γ ij ≈12.5 meV for the mid-infrared transition and Γ ij ≈4 meV for the THz transition, we obtain | χ (2) |≈22 nm V −1 and | χ (2) |≈10 nm V −1 at the alignment bias field corresponding to the operating point in the middle of the dynamic range for the active region presented in Fig. 2a , respectively. Device performance Structures were grown on semi-insulating InP substrates. Details of the growth sequence, processing steps and measurements are provided in the Methods section. Fabry–Perot devices produced broadband mid-infrared emission with a typical spectrum displayed in Fig. 3a . To produce narrowband THz sources, devices were processed as dual-colour surface DFB gratings for the mid-infrared lasers as shown in Fig. 3b , following the approach in ref. 22 . The gratings were written using electron beam lithography and were etched 130 nm deep into the upper waveguide cladding. The grating coupling coefficient, κ , was calculated to be ~25 cm −1 for both λ 1 and λ 2 pumps using COMSOL Multiphysics simulations based on the approach described in ref. 23 . 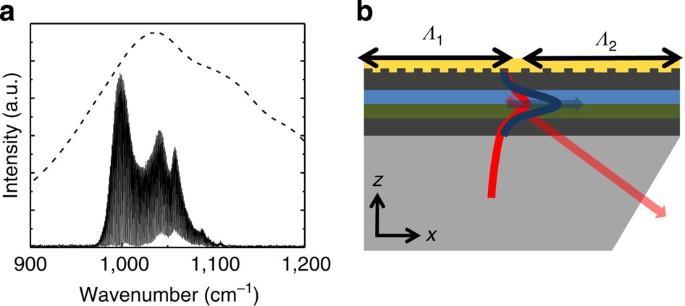Figure 3: Mid-infrared emission spectrum for Fabry–Perot lasers and distributed feedback device schematic. (a) Mid-infrared spectrum of a typical Fabry–Perot cavity device operated in pulsed mode at room temperature. Also shown is the electroluminescence (dashed line) from a 200-μm-diameter mesa at a current density of 7 kA cm−2that is indicative of the gain spectrum of our lasers. (b) Schematic of a dual-period surface DFB grating cavity with a Cherenkov waveguide. Coloured regions indicate top gold contact (yellow), active regions with non-linearity (blue and green), cladding layers (dark grey) and substrate (light grey). Cherenkov THz radiation (red) is emitted into the substrate. Dual-colour lasers presented in this paper had an approximately equal length of gratings sectionsΛ1andΛ2. Figure 3: Mid-infrared emission spectrum for Fabry–Perot lasers and distributed feedback device schematic. ( a ) Mid-infrared spectrum of a typical Fabry–Perot cavity device operated in pulsed mode at room temperature. Also shown is the electroluminescence (dashed line) from a 200-μm-diameter mesa at a current density of 7 kA cm −2 that is indicative of the gain spectrum of our lasers. ( b ) Schematic of a dual-period surface DFB grating cavity with a Cherenkov waveguide. Coloured regions indicate top gold contact (yellow), active regions with non-linearity (blue and green), cladding layers (dark grey) and substrate (light grey). Cherenkov THz radiation (red) is emitted into the substrate. Dual-colour lasers presented in this paper had an approximately equal length of gratings sections Λ 1 and Λ 2 . Full size image Room-temperature performance results are presented in Fig. 4 for a 1.7-mm-long × 25-μm-wide ridge laser with uncoated facets. The mid-infrared emission spectrum, collected at the laser pump current providing the maximum mid-infrared power output, is shown in Fig. 4a inset. The laser operated dual-wavelength emission at λ 1 =8.93 μm and λ 2 =10.14 μm over the entire dynamic range with a better-than 20 dB side-mode suppression ratio. Some additional peaks are located in the mid-infrared spectra at around 9.5 μm for this particular device and are 10 dB lower in power compared with the pumps. We note that these peaks may likely be eliminated if antireflective coatings are applied to the laser facets, which was not done to our devices. Other devices have no such ‘parasitic’ peaks (see Fig. 5 ). The L–I and V–I characteristics for the mid-infrared power output is displayed in Fig. 4a . The threshold current density was approximately the same as that of Fabry–Perot devices fabricated with the same wafer, indicating that the grating introduced negligible waveguide loss for the pumps. The corresponding THz spectrum is shown in Fig. 4b . The inset shows a side-mode suppression ratio better than 25 dB. 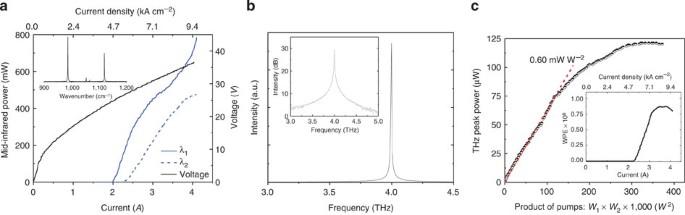Figure 4:Performance ofa 4-THz source. Spectral performance of a 1.70-mm-long × 25-μm-wide dual-period DFB grating device at room temperature. (a) Mid-infrared pump performance. Peak power (blue lines, bottom and left axis) and voltage (black line, bottom and right axis) versus current density. Mid-infrared power data is corrected for measured 70% mid-infrared collection efficiency of our setup. Mid-infrared emission spectrum of the device at current density of 9 kA cm−2(inset). (b) Corresponding THz emission spectrum taken at 9 kA cm−2. The same spectrum in logarithmic scale (inset). (c) THz peak power output versus the product of peak mid-infrared pump powers. THz output wall-plug efficiency versus current (inset). Figure 4c plots THz power output versus the product of the two mid-infrared pump powers. Nearly 120 μW of THz power output was recorded in a simple, two-parabolic-mirror setup without any correction for collection efficiency. A linear increase of THz power is observed with a 0.6 mW W −2 conversion efficiency, more than an order of improvement over Cherenkov DFG–QCLs with non-optimized waveguide structures [12] , [13] . The inset in Fig. 4c plots the THz output wall-plug efficiency as a function of current over the dynamic range of the device. A maximum efficiency of 0.9 × 10 −6 is observed at the device rollover point. Figure 4: Performance of a 4-THz source. Spectral performance of a 1.70-mm-long × 25-μm-wide dual-period DFB grating device at room temperature. ( a ) Mid-infrared pump performance. Peak power (blue lines, bottom and left axis) and voltage (black line, bottom and right axis) versus current density. Mid-infrared power data is corrected for measured 70% mid-infrared collection efficiency of our setup. Mid-infrared emission spectrum of the device at current density of 9 kA cm −2 (inset). ( b ) Corresponding THz emission spectrum taken at 9 kA cm −2 . The same spectrum in logarithmic scale (inset). ( c ) THz peak power output versus the product of peak mid-infrared pump powers. THz output wall-plug efficiency versus current (inset). 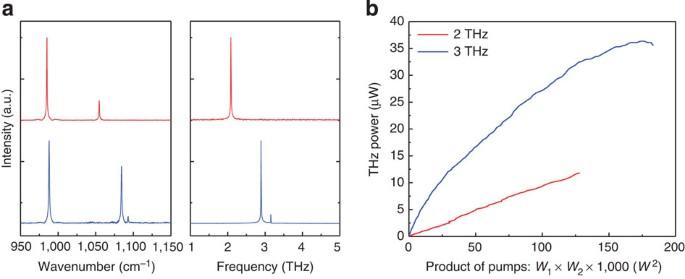Figure 5: Performance of 2 and 3 THz sources. Performance of 2 THz (red line) and 3 THz (blue line) sources. (a) Mid-infrared and THz spectral performance taken with a 0.2 cm−1resolution. (b) THz peak power output versus the product of mid-infrared pump powers. Full size image Figure 5: Performance of 2 and 3 THz sources. Performance of 2 THz (red line) and 3 THz (blue line) sources. ( a ) Mid-infrared and THz spectral performance taken with a 0.2 cm −1 resolution. ( b ) THz peak power output versus the product of mid-infrared pump powers. Full size image We also fabricated devices with mid-infrared DFB gratings designed for a pump frequency separation at 2 and 3 THz. The room temperature mid-infrared and THz emission spectra of these devices are shown in Fig. 5a and the THz power as a function of the product of the mid-infrared pump powers is shown in Fig. 5b . The 2 THz source produced nearly 12 μW of power with a constant 0.09 mW W −2 conversion efficiency and the 3 THz source generated 36 μW of power with a conversion efficiency of 0.4 mW W −2 at low bias. 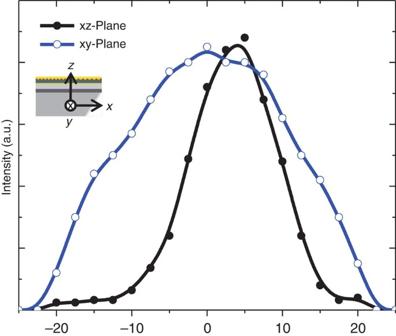Figure 6:THz far-field emission profile of a 4-THz device. Far-field THz emission profile in horizontal and vertical plane for the device. Angle of emission with respect to laser facets (degrees). THz far-field profile Figure 6 displays the far-field profile taken at the maximum THz power output for the 4 THz devicediscussed above. The bolometer was placed 15 cm away from the sample and was swept in the planes indicated in the figure inset. A narrow-emitting field 4° above normal incidence is obtained in the xz -plane. Directional THz output is a natural consequence of the Cherenkov emission process, which results in the whole polished substrate facet acting as THz emitter. In that regard, our Cherenkov THz–DFG sources are conceptually similar to THz QCLs with plasmatic collimators that make the whole substrate facet to act as THz emitter [24] . The maximum intensity is measured at +4°, which corresponds to an emission angle of ~21° in the substrate, in agreement with theoretical expectations. We note that the THz radiation emission angle can be adjusted by an appropriate choice of the substrate polish angle [12] . Higher THz beam divergence is observed in the xy plane, which is expected as the ridge width in our devices is only 25 μm. Figure 6: THz far -field emission profile of a 4-THz device. Far-field THz emission profile in horizontal and vertical plane for the device. Angle of emission with respect to laser facets (degrees). Full size image Broadband tuning with an EC Cherenkov DFG scheme allows for efficient extraction of THz radiation along the whole length of the QCL waveguide at any THz frequency [12] . As mid-infrared frequencies in a QCL can be tuned well over 5 THz [15] , [16] and optical non-linearity for intracavity THz DFG is not expected to change significantly over several THz of tuning [17] , Cherenkov DFG–QCLs are uniquely suited to be operated as broadly tunable THz sources for applications such as spectroscopy, microscopy and drug or explosives detection. High performance of the Cherenkov DFG–QCL chips reported here allowed us to demonstrate, for the first time, an EC DFG–QCL system, which is similar in mechanical design and operation to highly successful widely tunable mid-infrared EC QCL systems [15] , [25] . A schematic of the setup is shown in Fig. 7a . Primary system components include a 4-mm-diameter molded Chalcogenide glass plano-convex lens with a numerical aperture of 0.84 and a broadband antireflection coating in 8–12 μm and a gold-coated, 10.6-μm-wavelength-blazed grating with 150 groves per mm. We used a 1.7-mm-long, 22-μm-wide ridge waveguide Cherenkov DFG–QCL device, which contained a single period DFB grating over nearly the entire length of its waveguide. The grating parameters and processing was identical to that use for our single-mode THz DFG–QCL devices described earlier. This time, however, the grating period was kept constant to provide feedback at the mid-infrared wavelength of λ 1 =10.30 μm. The EC was then used to tune the lasing wavelength of the second mid-infrared pump from λ 2 =8.6–9.8 μm. The laser facets were left uncoated for this proof-of-concept demonstration. 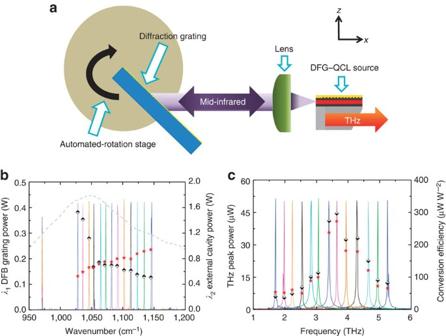Figure 7: Broadband tuning with an EC setup. (a) Schematic of the EC system operated in the Littrow configuration. (b) Mid-infrared spectra taken with a 0.2-cm−1resolution. The electroluminescence spectrum (grey, dashed line) displaying the gain bandwidth of the active region. Also shown are the power of the tunable-wavelengthλ2pump (red star, bottom and right axes) and that of the fixed-wavelengthλ1pump (black–white diamond, bottom and left axes) as a function ofλ2pump frequency. (c) Corresponding THz spectrum displaying a tuning bandwidth of 3.55 THz for our proof-of-concept EC system. The THz power (red star, bottom and left axes) and conversion efficiency (black–white diamond, bottom and right axes) is shown for each wavelength. Figure 7: Broadband tuning with an EC setup. ( a ) Schematic of the EC system operated in the Littrow configuration. ( b ) Mid-infrared spectra taken with a 0.2-cm −1 resolution. The electroluminescence spectrum (grey, dashed line) displaying the gain bandwidth of the active region. Also shown are the power of the tunable-wavelength λ 2 pump (red star, bottom and right axes) and that of the fixed-wavelength λ 1 pump (black–white diamond, bottom and left axes) as a function of λ 2 pump frequency. ( c ) Corresponding THz spectrum displaying a tuning bandwidth of 3.55 THz for our proof-of-concept EC system. The THz power (red star, bottom and left axes) and conversion efficiency (black–white diamond, bottom and right axes) is shown for each wavelength. Full size image Mid-infrared spectra and power of the mid-infrared pumps at λ 1 and λ 2 are displayed in Fig. 7b for different grating angles. The spectra were taken at room temperature at a pump current density 8 kA cm −2 , close to the rollover point. The corresponding THz spectrum shown in Fig. 7c displays recorded emission spectra of the EC DFG–QCL system for operation between 1.70 and 5.25 THz. Single-frequency emission with a side-mode suppression ratio of better than 15 dB is observed for nearly all THz signals with the exception for the THz emission at the periphery of the systems tuning range that have parasitic lasing peaks in the mid-infrared spectrum corresponding to the active region gain peak. Antireflection coating for the mid-infrared facets that are used for high-performance mid-infrared EC QCLs [15] , [25] is expected to suppress this parasitic lasing and improve the spectral purity. The power and conversion efficiency at each THz wavelength is also plotted in Fig. 7c . At 3.6 THz, a maximum power and conversion efficiency of 40 μW and 0.3 mW W −2 , respectively, is measured in general agreement with the conversion efficiency of DFB DFG–QCLs operating at 3 and 4 THz near the rollover point, cf. Figs 5b and 4c , respectively. DFG–QCLs reported here have demonstrated by far the highest power output and conversion efficiency for THz DFG–QCL sources. It is worth noting that all DFG–QCLs reports so far [10] , [11] , [12] , [13] , [14] used at least a 50% ‘collection efficiency’ correction factor for THz power, although this number is difficult to determine accurately. In contrast, the THz power data in this paper is collected using a simple two-parabolic-mirror setup and contains no ‘collection efficiency’ correction. Thus, for practical applications, the power and conversion efficiency improvements in the THz sources reported here are even more significant. Remarkably and importantly, a very considerable room for performance improvement still exists, even for the current device design. In particular, the lasers were grown on a 350-μm-thick semi-insulating InP substrates with the output facet polished at 30° for devices reported above. From simple geometrical considerations, assuming θ C =20° and a substrate polish angle of 30°, only the Cherenkov radiation generated within 1.15 mm from the exit facet can be outcoupled, and radiation generated further away undergoes multiple reflections and is eventually absorbed in the substrate (see Fig. 1a ). We have measured an absorption coefficient of α =15 cm −1 at 4 THz for the substrates used in our devices and this number matches well with other sources [22] . For our particular case, 50% of power in the Cherenkov wave generated from the 1.15-mm-long section and propagating towards the output facet is lost to absorption. Furthermore, the output facet in our devices does not have any antireflection coatings and transmits only an estimated 72% of incident THz power. Finally, we note that Cherenkov waves are generated towards both front and back facet of the laser, and we only collect the wave that propagates towards the front facet. Thus, for a 1.7-mm-long DFB device described in the text, only 12% of the total generated THz power in Cherenkov waves is being outcoupled. The theoretical estimate for the conversion efficiency in our devices may be obtained from Fig. 1b , using a 1.15-mm-long section of the laser waveguide that contribute to the outcoupled Cherenkov wave, and correcting the Cherenkov wave power for 50% absorption loss in the substrate and 28% reflection loss at the facet. We obtain the value of 2.65 mW W −2 , close to that measured experimentally. The wall-plug efficiency of the 4 THz DFG–QCL source peaks at ~0.9 × 10 −6 near rollover point (see Fig. 4c , inset). In comparison, THz QCLs systems integrated with pulsed-tube cryorefrigerators [26] or Stirling cryocoolers [27] have a wall-plug efficiency of about 10 −5 , once taking into account the power consumption of the cooling system. Clearly, a cryocooler also adds to the system size and complexity. Given the rapid progress of THz DFG–QCL technology, one may expect significant improvement wall-plug efficiency in future generation of sources. Manley–Rowe relations may be viewed as the fundamental limit on wall-plug efficiency for THz DFG systems. From this perspective, given the current record values for room-temperature, pulsed-operation wall-plug efficiency of mid-infrared QCLs of 27% at λ ~5 μm [28] and 6% at λ ~10 μm [29] , we obtained the Manley–Rowe-limited wall-plug efficiency value of ~10 −2 for 4 THz generation in DFG–QCLs at room temperature. Different configurations may be considered for more efficient Cherenkov wave outcoupling, including using grating structures or external optical components (prisms) for efficient outcoupling of both left- and right-going Cherenkov waves, especially for long (>2 mm) devices. Additional improvements that may be implemented in the future include optimizing the quantum design of the active regions to possess higher optical non-linearity and to reach maximum non-linearity at the rollover point close to the peak of the mid-infrared pump power. Device growth and fabrication The laser structure was grown by molecular beam epitaxy on a 350-μm-thick semi-insulating InP substrate. The growth commenced with a 200-nm-thick InGaAs current injection layer (Si, 7 × 10 17 cm −3 ), followed by a 3-μm-thick InP lower cladding doped (Si, 1.5 × 10 16 cm −3 ). The active region was grown next and made with a InGaAs/InAlAs heterostructure lattice matched to InP. It is comprised of 33 repetitions of the λ 1 =9.20 μm design followed by 33 repetitions of the λ 2 =8.20 μm design. The layer sequence of the λ 1 =9.20 μm design, starting with the injection barrier, is 39 /22/ 8 /60/ 9 /59/ 10 /52/ 13 /43/ 14 /38/ 15 /36/ 16 /34/ 19 /33/ 23 /32/ 25 /32 / 29 /31, and for the λ 2 =8.20 μm design is 43 /18/ 7 /55/ 9 /53/ 11 /48/ 14 /37/ 15 /35/ 16 /33/ 18 /31/ 20 /29/ 24 /29/ 26 /27 / 30 /27, where the layer thicknesses are in angstroms, bold numbers indicate barriers, and underlined numbers indicate regions doped with Si to n =2 × 10 17 cm −3 . The top cladding layer consists of a 3-μm-thick InP (Si, 1.5 × 10 16 cm −3 ), followed by a 100-nm-thick InP layer (Si, 3 × 10 18 cm −3 ) and terminated with a 10-nm-thick InGaAs contact layer (Si, 2 × 10 19 cm −3 ). Samples were processed into dry-etched ridge waveguides via inductive plasma etching. Ridge widths varied between 18 and 40 μm. The sidewalls of the ridges were insulated with a 400-nm-thick layer of silicon nitride, followed by Ti/Au (15 nm/800 nm) contact metallization. Given the insulating nature of the substrate, a lateral contact current injection scheme was employed. The wafer was cleaved into laser bars ~1- to 2-mm long. The 350-μm-thick InP substrate associated with the THz exit facet of the device was mechanically polished at a 30° angle for the THz Cherenkov wave outcoupling with Al 2 O 3 lapping film. Special care was taken to ensure that the laser waveguide facets are unaffected by polishing. Devices were then Indium soldered epi-side up onto copper holders and were wire bonded. Cherenkov wave modelling For the Cherenkov emission simulation, a slab-waveguide model was used as described in text. THz power of the Cherenkov wave was obtained by multiplying the wave power density (obtained from slab-waveguide simulations) by the ridge area of our devices. The values of the refractive indices for the waveguide layers were obtained by combining the table values of the refractive indices of undoped semiconductor compounds with the Drude model that used a relaxation time constant τ =10 −13 s to account for the free-carrier contribution. The refractive indices of undoped Al 0.48 In 0.52 As and In 0.53 Ga 0.47 As compounds in the waveguide core are calculated using the linear interpolation between the data for the binary compounds. We note that this approach is known to work well in the mid-infrared; however, it may not be very accurate in THz because of the proximity of the Reststrahlen band and the strong dependence of the optical phonon energies on the material composition. Experimental measurements All measurements were done at room temperature, in pulsed mode using 100 ns current pulses at a 5-kHz repetition frequency. Spectral emission of the mid-infrared and THz beams was measured using a Fourier-transform infrared spectrometer. Appropriate filters were used to separate the mid-infrared and THz signals. A helium-cooled silicon bolometer and deuterated L -alanine doped triglycine sulphate detector were used for the THz and mid-infrared spectral measurements, respectively. The output power of devices was measured with an off-axis parabolic-mirror setup in a nitrogen-purged environment. Calibrated thermopile and pyroelectric detectors were used to measure power for the mid-infrared beams, and a Golay-cell calibrated helium-cooled silicon bolometer for the THz signal. The mid-infrared data presented in the paper is corrected for a measured 70% collection efficiency of our setup. The THz data is not corrected for collection efficiency. How to cite this article: Vijayraghavan, K. et al . Broadly tunable terahertz generation in mid-infrared quantum cascade lasers. Nat. Commun. 4:2021 doi: 10.1038/ncomms3021 (2013).